Activating CAR and β-catenin induces uncontrolled liver growth and tumorigenesis Aberrant β-catenin activation contributes to a third or more of human hepatocellular carcinoma (HCC), but β-catenin activation alone is not sufficient to induce liver cancer in mice. Differentiated hepatocytes proliferate upon acute activation of either β-catenin or the nuclear xenobiotic receptor CAR. These responses are strictly limited and are tightly linked, since β-catenin is activated in nearly all of the CAR-dependent tumours generated by the tumour promoter phenobarbital. Here, we show that full activation of β-catenin in the liver induces senescence and growth arrest, which is overcome by combined CAR activation, resulting in uncontrolled hepatocyte proliferation, hepatomegaly and rapid lethality despite maintenance of normal liver function. Combining CAR activation with limited β-catenin activation induces tumorigenesis, and the tumours share a conserved gene expression signature with β-catenin-positive human HCC. These results reveal an unexpected route for hepatocyte proliferation and define a murine model of hepatocarcinogenesis with direct relevance to human HCC. The incidence of hepatocellular carcinoma (HCC), the fifth most common cancer worldwide, has more than tripled in the United States over the last 20 years, while 5-year survival remains below 12%. Although positive outcomes have recently been obtained with the tyrosine kinase inhibitor sorafenib, the limited effectiveness of standard chemotherapeutic approaches makes HCC the third leading cause of cancer-related mortality [1] , [2] . The Wnt/β-catenin signalling pathway regulates key aspects of mammalian cell biology, including proliferation, differentiation and cell fate determination. Under normal circumstances, β-catenin is phosphorylated by GSK3β and quickly degraded by the ubiquitin/proteasome pathway. Aberrant Wnt pathway activation via β-catenin stabilization is a critical contributor to many different cancers, including a large fraction of hepatocellular carcinomas [3] , [4] . However, liver-specific activation of β-catenin in mice is not sufficient to induce spontaneous liver tumours [5] , [6] , [7] , [8] . Deregulated β-catenin can activate p53 and trigger an anti-proliferative response in mouse embryo fibroblasts, with prolonged β-catenin activation resulting in growth arrest [9] . Wnt/β-catenin activation also induces senescence in fibroblasts and in mouse skin, and a p53-dependent DNA damage response and senescence in both mesenchymal stem cells and the gut [10] , [11] , [12] . Thus, oncogene-induced senescence may block tumorigenesis in response to β-catenin activation. CAR (Constitutive Androstane Receptor, NR1I3) is a primary regulator of drug metabolism and detoxification. In addition to inducing hepatic drug metabolism, acute CAR activation results in rapid, but transient and strictly limited liver growth. CAR activators, including phenobarbital (PB) and the much more potent, specific and persistent agonist TC (TCPOBOP; 1,4-Bis[2-(3,5- dichloropyridyloxy)]benzene), are both non-genotoxic carcinogens and liver tumour promoters, and CAR is required for their tumorigenic effects [13] , [14] , [15] , [16] . A tight functional interaction between CAR and β-catenin was revealed by the striking observation that 80% or more of the liver tumours produced in the widely used carcinogen/initiator (diethylnitrosamine) plus promoter (PB) mouse model of hepatocarcinogenesis carry activating mutations in β-catenin [17] , [18] . In contrast, β-catenin activation was not observed in tumours induced by diethylnitrosamine alone [17] . Consistent with this, PB treatment selects for a β-catenin-positive cell population in the c-Myc/TGF-α transgenic mouse model of HCC, and the activation of β-catenin provides proliferative and invasive advantages in this model [19] . In addition, liver-specific loss of β-catenin impairs the induction of CAR-mediated drug-metabolizing enzymes and hepatocyte proliferation in male mice (although the proliferative effect was not observed in female mice), and eliminates the promotion activity of PB [20] , [21] , [22] , [23] . These results suggest a unique cooperation between CAR and β-catenin in liver tumorigenesis. In this study, we explore their functional synergy in vivo using pharmacologic and genetic tools. β-Catenin is activated by adenoviral Cre in previously described mice homozygous or heterozygous for paired loxP sites flanking β-catenin exon 3 ( ctnnb1 loxP(ex3) ), which contains the phosphorylation sites targeting intracellular β-catenin for degradation [5] , [24] . Treating mice with a single dose of the potent and persistent agonist TC activates hepatic CAR over a time course of months. We found that full activation of both pathways results in sustained hepatocyte proliferation and rapid death from hepatomegaly. Finally, long-term pharmacologic CAR activation together with partial β-catenin activation is sufficient to induce tumours that share a conserved gene expression signature with β-catenin-positive human HCC. Activation of CAR and β-catenin induces liver growth β-Catenin has been reported to act as a nuclear receptor coactivator [25] , [26] , providing a simple potential explanation for the observed functional synergy of CAR and β-catenin. However, extensive studies showed no evidence for direct transcriptional interactions. Thus, we found no effects of β-catenin expression on CAR transactivation, or vice versa, in transiently transfected liver cell lines ( Supplementary Fig. 1a ). We did not observe any change in β-catenin signalling in wild-type (WT) or CAR −/− mice treated with TC or PB, as indicated by expression of β-catenin and its downstream transcriptional targets glutamine synthetase (GS) and Axin2 ( Supplementary Fig. 1b ). These results indicate that neither of the transcription factors directly modulates the transcriptional output of the other. To pursue potential functional interactions of CAR and β-catenin in more depth in vivo , we used mice carrying loxP sites flanking β-catenin exon 3 ( ctnnb1 loxP(ex3)/loxP(ex3) ), which contains the phosphorylation sites targeting intracellular β-catenin for degradation. As previously described [5] , acute deletion of this exon by Ad-Cre (Cre expressing adenovirus) infection activates β-catenin specifically in the liver. We genetically activated β-catenin by infecting homozygous ctnnb1 loxP(ex3)/loxP(ex3) mice with a high titer (10 9 p.f.u.) of Ad-Cre or Ad-Ctrl (Control) adenoviruses and also activated CAR by treating them at the same time with a single dose of TC or vehicle. Mice were killed 1–4 weeks after treatment. As expected, liver size increased acutely in response to treatment by either TC or Ad-Cre alone, but growth stopped after either 1 or 2 weeks, respectively. In striking contrast, growth in the doubly activated TC plus Ad-Cre treatment group was unconstrained, with liver weight (LW) reaching 25% of total body weight (BW) at 4 weeks ( Fig. 1a,b and Supplementary Data 1 ). Mortality was observed in the TC plus Ad-Cre-treated group starting at 3 weeks after the initiation of both treatments. We attribute this lethal phenotype to hepatomegaly, since a panel of serum indicators showed normal liver function ( Supplementary Fig. 2 ). Ki67 staining confirmed a dramatic increase in hepatocyte proliferation in the doubly activated livers ( Fig. 1c and Supplementary Fig. 3 ). In accord with this, histology showed disorganized and enlarged liver cells in the doubly activated group ( Fig. 1c ). Immunohistochemical analysis revealed nuclear localization of β-catenin in both Ad-Cre and Ad-Cre plus TC groups ( Fig. 1c ). Expression of the β-catenin target gene GS is restricted to the perivenous region of the hepatic lobule in control and TC-treated mice, as expected, but was dramatically increased throughout the lobule in the Ad-Cre-treated groups ( Fig. 1c ). 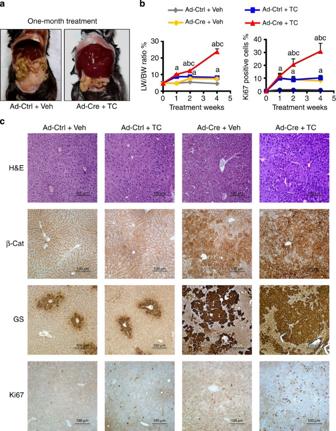Figure 1: Synergistic induction of liver growth by combined β-catenin and CAR activation. Homozygousctnnb1loxP(ex3)/loxP(ex3)mice were infected with 109pfu of Ad-Ctrl or Ad-Cre adenoviruses via tail vein injection in a single experiment. Mice were treated with a single dose of TC or vehicle and analysed at the indicated time points. (a) Enlarged liver in β-catenin and CAR doubly activated mice. (b) Liver size and proliferation were assessed by liver/body weight ratio and ki67 staining (n=4 to 8; One-way ANOVA was used for statistical analysis and a/b/c comparisons are significant (detailedPvalue shown inSupplementary Data 1); (a): versus Ad-Ctrl+Veh; (b): versus Ad-Ctrl+TC; (c): versus Ad-Cre+Veh; data are represented as mean±s.e.m.). (c) Haematoxylin and eosin (H&E) staining for liver histology immunostaining of β-catenin (β-cat), glutamine synthetase (GS) and Ki67 were assessed at 1 month after treatment (Scale bar, 100 μm). Figure 1: Synergistic induction of liver growth by combined β-catenin and CAR activation. Homozygous ctnnb1 loxP(ex3)/loxP(ex3) mice were infected with 10 9 pfu of Ad-Ctrl or Ad-Cre adenoviruses via tail vein injection in a single experiment. Mice were treated with a single dose of TC or vehicle and analysed at the indicated time points. ( a ) Enlarged liver in β-catenin and CAR doubly activated mice. ( b ) Liver size and proliferation were assessed by liver/body weight ratio and ki67 staining ( n =4 to 8; One-way ANOVA was used for statistical analysis and a/b/c comparisons are significant (detailed P value shown in Supplementary Data 1 ); (a): versus Ad-Ctrl+Veh; (b): versus Ad-Ctrl+TC; (c): versus Ad-Cre+Veh; data are represented as mean±s.e.m.). ( c ) Haematoxylin and eosin (H&E) staining for liver histology immunostaining of β-catenin (β-cat), glutamine synthetase (GS) and Ki67 were assessed at 1 month after treatment (Scale bar, 100 μm). Full size image Full activation of both β-catenin and CAR was confirmed by induction of their target genes (Cyp2b10 and Gadd45β for CAR; GS and Axin2 for β-catenin ( Fig. 2a ). Cyclin D1 and c-Myc [27] , [28] were induced in the singly TC-treated or Ad-Cre-infected mice, with an additive effect of the combined activation of both CAR and β-catenin. Two-way analysis of variance (ANOVA) revealed that there was a significant interaction (F=5.267, P =0.0406) between β-catenin and CAR activation in inducing Cyclin D1 expression ( Supplementary Data 2 ). Interestingly, the HCC-associated genes Igf2 and Sox4 were induced in the TC-treated groups, while the HCC marker AFP was induced in Ad-Cre-treated mice ( Fig. 2a ). Yap is also essential for the proliferation of a number of β-catenin-positive cancer cell lines [29] . Here, we observed increased expression of the Yap targets Birc5 and Ccne1 and 2 in response to β-catenin activation in both Cre and Cre plus TC groups ( Fig. 2b ). Yap phosphorylation was decreased, indicating Hippo pathway inactivation and Yap activation, in the doubly activated livers at 1 month ( Fig. 2b ). However, we did not observe Yap dephosphorylation in response to activation of β-catenin alone, or in the doubly activated livers at 2 weeks. Thus, the Hippo pathway may also contribute to the later stages of the combined effects of β-catenin and CAR. 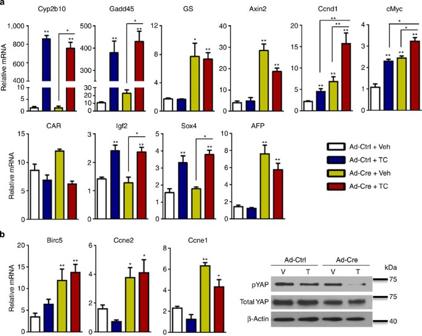Figure 2: Gene expression induced by combined β-catenin and CAR activation. (a) Liver samples were collected from the mice described inFig. 1. Total RNA was extracted and gene expression was measured by quantitative PCR with reverse transcription (qRT–PCR;n=4 to 5; *P<0.05; data are represented as mean±s.e.m.). (b) Gene expression in Hippo signaling pathway was analysed by qRT–PCR and western blot. (n=4–5; *P<0.05, **P<0.01; data are represented as mean±s.e.). Student’st-test was used for statistical analysis. Gene expression is repeated twice for all the experiments. Figure 2: Gene expression induced by combined β-catenin and CAR activation. ( a ) Liver samples were collected from the mice described in Fig. 1 . Total RNA was extracted and gene expression was measured by quantitative PCR with reverse transcription (qRT–PCR; n =4 to 5; * P <0.05; data are represented as mean±s.e.m.). ( b ) Gene expression in Hippo signaling pathway was analysed by qRT–PCR and western blot. ( n =4–5; * P <0.05, ** P <0.01; data are represented as mean±s.e.). Student’s t -test was used for statistical analysis. Gene expression is repeated twice for all the experiments. Full size image CAR activation overcomes β-catenin-induced senescence Activation of Wnt/β-catenin signalling can engage oncogene-induced senescence both in vitro and in vivo , and this p53-mediated growth control mechanism can be overcome by ablation of p53 or its target gene p21 (refs 9 , 10 , 11 ). Senescent cells produce increased amounts of inflammatory cytokines, and previous results indicated that activation of hepatic β-catenin signalling induces such an inflammatory signature [30] , [31] . Thus, we hypothesized that induction of senescence could limit liver growth following β-catenin activation. Histologically, Ad-Cre livers showed recruitment of inflammatory cells, a typical signature of senescence that was reversed by TC treatment in the double activation group ( Fig. 3a ). Inflammatory cytokines such as Csf1, Mcp1, Cxcl10 and Icam were upregulated in the Ad-Cre livers, but not in the doubly activated Ad-Cre plus TC livers ( Fig. 3c ). Increased expression of the primary marker SA-β-galactosidase in hepatocytes strongly confirmed the senescent response to β-catenin activation, and this was also suppressed by combined activation of CAR ( Fig. 3a,b ). As predicted from its association with oncogene-induced senescence, p53 was induced in the Ad-Cre-treated group, along with its growth inhibitory target genes p21 and p27 ( Fig. 3d,e ). As expected, two-way ANOVA analysis shows significant interaction between β-catenin and CAR activation in regulating many genes including p21, Mcp1, Cxcl10 and Csf ( Supplementary Data 3 ). 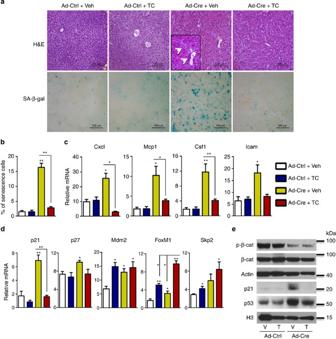Figure 3: CAR activation suppresses β-catenin-induced p53 response and cellular senescence. Ctnnb1loxP(ex3)/loxP(ex3)mice were infected with a high titer (109p.f.u.) of Ad-Ctrl or Ad-Cre viruses, and treated with a single dose of TC or vehicle. The experiment was repeated twice. Mice were killed at 2 weeks and assessed for: (a) haematoxylin and eosin (H&E) staining and SA-β-gal staining. White arrows in × 40 inset indicate inflammatory infiltrates in Ad-Cre plus vehicle-treated livers (Scale bar, 100 μm). (b) Quantification of β-gal positive senescent hepatocytes in indicated treatment groups. (c) The expression of inflammatory cytokines were measured by quantitative PCR with reverse transcription (qRT–PCR). Gene expression was repeated three times. (d) mRNA expression of mdm2, p21, p27, FoxM1 and Skp2 were measured by qRT–PCR. Gene expression was repeated three times. (e) Phospho- and total β-catenin, p53 and its target p21 expression were assessed by western blot. Protein expression was repeated three times. ((b–e):n=4–5; Student’st-test was used for statistical analysis, *P<0.05; data are represented as mean±s.e.m.). Figure 3: CAR activation suppresses β-catenin-induced p53 response and cellular senescence. Ctnnb1 loxP(ex3)/loxP(ex3) mice were infected with a high titer (10 9 p.f.u.) of Ad-Ctrl or Ad-Cre viruses, and treated with a single dose of TC or vehicle. The experiment was repeated twice. Mice were killed at 2 weeks and assessed for: ( a ) haematoxylin and eosin (H&E) staining and SA-β-gal staining. White arrows in × 40 inset indicate inflammatory infiltrates in Ad-Cre plus vehicle-treated livers (Scale bar, 100 μm). ( b ) Quantification of β-gal positive senescent hepatocytes in indicated treatment groups. ( c ) The expression of inflammatory cytokines were measured by quantitative PCR with reverse transcription (qRT–PCR). Gene expression was repeated three times. ( d ) mRNA expression of mdm2, p21, p27, FoxM1 and Skp2 were measured by qRT–PCR. Gene expression was repeated three times. ( e ) Phospho- and total β-catenin, p53 and its target p21 expression were assessed by western blot. Protein expression was repeated three times. (( b – e ): n =4–5; Student’s t -test was used for statistical analysis, * P <0.05; data are represented as mean±s.e.m.). Full size image A recent study showed that activating β-catenin via inactivation of Apc induces liver inflammation through direct targeting of proinflammatory target genes in hepatocytes, particularly the chemokine-like chemotactic factor leukocyte cell-derived chemotaxin 2 (Lect2) [31] , and we also observed Lect2 induction in the Ad-Cre livers ( Supplementary Fig. 4a ). This suggests the possibility that concomitant CAR activation might suppress inflammation via inhibition of Lect2 induction. In contrast, CAR activation also induces Lect2 and this induction is CAR dependent ( Supplementary Fig. 4b ). However, we did not observe significant induction of Lect2 mRNA in the tumours from our mouse model ( Supplementary Fig. 4a ). Thus, suppression of Lect2 expression cannot account for the anti-inflammatory effects of combined CAR and β-catenin activation. We showed previously that CAR activation strongly suppresses p53 responses by directly inducing its primary inhibitor, Mdm2 (ref. 14 ). p53 also induces Mdm2 in a well-known negative feedback loop, and Mdm2 was induced to comparable levels in both the singly activated groups at 2 weeks ( Fig. 3d ). Importantly, however, TC treatment activates such primary CAR targets within hours and persists for months, while p53 induction is a secondary consequence of the growth response to β-catenin activation. Thus, the prior CAR dependent induction of Mdm2 should override the later p53 response in the doubly activated livers. As expected, p53 protein levels were decreased in the doubly activated livers relative to the singly β-catenin-activated livers, and the induction of its downstream target p21 was also reversed ( Fig. 3d,e ). In addition to Mdm2, CAR also induces the transcription factor FoxM1, a key mediator of CAR-induced liver growth [32] . Overexpression of FoxM1 is associated with the development and progression of many cancers including lung, prostate, pancreatic, glioblastoma and HCC [33] , [34] , [35] . This pathway is also relevant to senescence, because overexpression of FoxM1 suppresses p53 and p21 expression [36] , [37] , [38] , and its downstream target Skp2 also suppresses expression of the cell cycle inhibitors p21 and p27 (refs 39 , 40 , 41 ). FoxM1 and Skp2 were induced by TC treatment, as expected ( Fig. 3d ). β-catenin activation also increased FoxM1 mRNA, and the highest levels of both FoxM1 and Skp2 were observed in the doubly activated livers. Consistent with this, the Skp2 target p21 was suppressed in the doubly treated group, indicating that the FoxM1-Skp2 activation may also contribute to the suppression of senescence caused by β-catenin. Overall, we conclude that oncogene-induced senescence limits the growth response to acute β-catenin activation in the liver, and that CAR activation can overcome this blockade. Long-term activation of CAR and β-catenin induces HCC The early mortality induced by full β-catenin and CAR activation in the ctnnb1 loxP(ex3)/loxP(ex3) mice prevented studies of tumorigenesis. We, therefore, focused on mice heterozygous for the loxP flanked β-catenin allele ( ctnnb1 wt/loxP(ex3) ; wt: wild type), which do not show acute growth or induction of c-Myc or Cyclin D1 in response to high titre Ad-Cre infection. We infected heterozygous ctnnb1 wt/loxP(ex3) mice with high titres of Ad-Ctrl or Ad-Cre viruses plus a single dose of TC or vehicle, and followed them without further treatment for up to 8 months. Knockout of exon 3 at 2 weeks and 8 months was confirmed by PCR ( Supplementary Fig. 5a ). The activation of both β-catenin and CAR was confirmed by appropriate target gene expression at 2 weeks ( Fig. 4a ). No mortality was observed throughout the experiment. At 8 months, large tumours were observed only in the mice treated with both Ad-Cre and TC; neither TC treatment alone, as expected for the C57BL/6 mouse strain, nor Ad-Cre-induced β-catenin activation induced liver tumorigenesis ( Fig. 4b ). To test the predicted CAR dependence of this mouse model, we crossed the ctnnb1 wt/loxP(ex3) mice with the CAR null allele to generate CAR −/− ; ctnnb1 wt/loxP(ex3) mice. We again treated the mice with Ad-Cre or Ad-Ctrl, with or without a single dose of TC. In these mice, Ad-Cre activation of β-catenin is maintained, but TC treatment does not activate CAR targets such as Cyp2b10 ( Fig. 4a ). Two-way ANOVA did not show significant interaction of CAR and β-catenin activation ( Supplementary Data 4 ). After 8 months, there was no tumorigenesis in the TC and Ad-Cre double-treated group, confirming the expected CAR dependence ( Table 1 ). 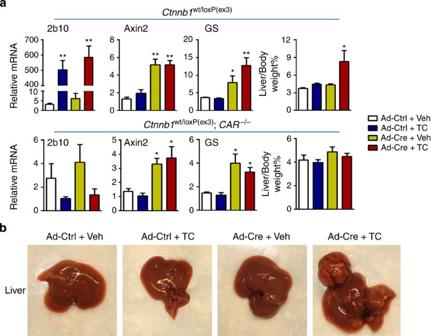Figure 4: Long-term activation of β-catenin plus CAR causes liver tumorigenesis. (a) Heterozygousctnnb1wt/loxP(ex3)mice andctnnb1wt/loxP(ex3);CAR−/−mice were infected with 109p.f.u. of Ad-Ctrl or Ad-Cre virus and treated with one dose of TC or vehicle treatment in a single experiment. Two weeks later, four mice from each group were killed and liver total RNA was extracted. Gene expression was analysed for β-catenin and CAR activation (n=4–5; Student’st-test was used for statistical analysis, *P<0.05; data are represented as mean±s.e.m.). Gene expression was repeated three times. Eight months later, liver tumorigenesis was assessed in different groups. Liver weight and body weight ratios were analysed. (b) Macroscopic liver appearance. Figure 4: Long-term activation of β-catenin plus CAR causes liver tumorigenesis. ( a ) Heterozygous ctnnb1 wt/loxP(ex3) mice and ctnnb1 wt/loxP(ex3) ; CAR −/− mice were infected with 10 9 p.f.u. of Ad-Ctrl or Ad-Cre virus and treated with one dose of TC or vehicle treatment in a single experiment. Two weeks later, four mice from each group were killed and liver total RNA was extracted. Gene expression was analysed for β-catenin and CAR activation ( n =4–5; Student’s t -test was used for statistical analysis, * P <0.05; data are represented as mean±s.e.m.). Gene expression was repeated three times. Eight months later, liver tumorigenesis was assessed in different groups. Liver weight and body weight ratios were analysed. ( b ) Macroscopic liver appearance. Full size image Table 1 Tumour incidence for main Fig. 4 . Full size table The Ad-Cre plus TC tumours showed a typical HCC phenotype with peliosis ( Fig. 5 ). There was no staining of nuclear β-catenin or alteration in GS staining in the control or CAR-activated groups as expected, but GS expression was moderately elevated and a few cells still showed nuclear β-catenin in the Ad-Cre group. In contrast, the tumours in the TC/Ad-Cre doubly treated group showed increased nuclear and cytoplasmic expression of β-catenin, with marked induction of GS as well as HCC marker alpha-fetoprotein (AFP). Increased GS expression was confirmed by western blot ( Supplementary Fig. 5b ). High numbers of BrdU-positive cells confirmed the active proliferation of the tumour ( Fig. 5 ). Gene expression studies confirmed the induction of β-catenin target genes GS and Axin2 in the tumours of the doubly activated livers ( Fig. 6 ). CAR expression was not altered significantly, while elevated Cyp2b10 was maintained in TC- and TC/Ad-Cre-treated groups. As expected, the tumours showed increased Cyclin D1 and c-Myc expression, and they also expressed several known HCC-associated markers, including H19, Igf2, AFP and Sox4. Interestingly, and in accord with short-term treatment in the Ad-Cre plus TC-treated group, Mdm2, FoxM1 and Skp2 were also induced in the tumours, along with the Yap target Birc5 ( Fig. 6 ). 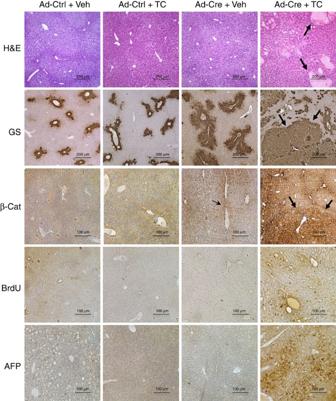Figure 5: Histology analysis of β-catenin plus CAR-induced liver tumours. Heterozygousctnnb1wt/loxP(ex3)mice were infected with 109p.f.u. of Ad-Ctrl or Ad-Cre virus and treated with one dose of TC or vehicle treatment in a single experiment. Eight months later, liver samples were collected for further analysis. Representative figures fromn=8–10 mice per group. Haematoxylin and eosin (H&E) staining shows relatively normal histology for control and singly activated livers. Ad-Cre+TC tumour histology shows cell crowding and empty structures, indicating peliosis (Scale bar, 200 μm). Immunostaining for β-catenin target glutamine synthetase (GS) (Scale bar, 200 μm) shows normal pericentral expression in both Ad-Ctrl-infected livers, increased expression in singly β-catenin-activated livers, and much more broad and uniform expression in the β-catenin and CAR doubly activated tumours. β-Catenin staining shows normal membrane expression in both Ad-Ctrl+Veh and Ad-Ctrl+TC livers. Ad-Cre+Veh group shows limited number of β-catenin-positive nuclei (arrows). Ad-Cre+TC group tumours show more consistent nuclear β-catenin staining. β-Catenin and CAR doubly activated tumours express the HCC marker alpha-fetoprotein and show increased proliferation by BrdU staining (Scale bar, 100 μm). Figure 5: Histology analysis of β-catenin plus CAR-induced liver tumours. Heterozygous ctnnb1 wt/loxP(ex3) mice were infected with 10 9 p.f.u. of Ad-Ctrl or Ad-Cre virus and treated with one dose of TC or vehicle treatment in a single experiment. Eight months later, liver samples were collected for further analysis. Representative figures from n =8–10 mice per group. Haematoxylin and eosin (H&E) staining shows relatively normal histology for control and singly activated livers. Ad-Cre+TC tumour histology shows cell crowding and empty structures, indicating peliosis (Scale bar, 200 μm). Immunostaining for β-catenin target glutamine synthetase (GS) (Scale bar, 200 μm) shows normal pericentral expression in both Ad-Ctrl-infected livers, increased expression in singly β-catenin-activated livers, and much more broad and uniform expression in the β-catenin and CAR doubly activated tumours. β-Catenin staining shows normal membrane expression in both Ad-Ctrl+Veh and Ad-Ctrl+TC livers. Ad-Cre+Veh group shows limited number of β-catenin-positive nuclei (arrows). Ad-Cre+TC group tumours show more consistent nuclear β-catenin staining. β-Catenin and CAR doubly activated tumours express the HCC marker alpha-fetoprotein and show increased proliferation by BrdU staining (Scale bar, 100 μm). 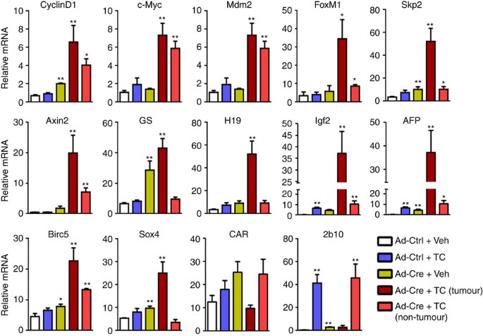Figure 6: Gene expression pattern in β-catenin plus CAR-induced liver tumours. Mice were treated as indicated inFig. 5. Liver samples from different groups were collected and total RNA was extracted for expression analysis. Gene expression was repeated two times. For the Ad-Cre plus TC mice, tumour (TC(T)) and normal non-tumour liver (TC(NT) samples were separated and processed for quantitative PCR with reverse transcription analysis (n=5; Student’st-test was used for statistical analysis, *P<0.05). Full size image Figure 6: Gene expression pattern in β-catenin plus CAR-induced liver tumours. Mice were treated as indicated in Fig. 5 . Liver samples from different groups were collected and total RNA was extracted for expression analysis. Gene expression was repeated two times. For the Ad-Cre plus TC mice, tumour (TC(T)) and normal non-tumour liver (TC(NT) samples were separated and processed for quantitative PCR with reverse transcription analysis ( n =5; Student’s t -test was used for statistical analysis, * P <0.05). Full size image We further confirmed the sufficiency of CAR and β-catenin activation for liver tumorigenesis by treating homozygous ctnnb1 loxP(ex3)/loxP(ex3) mice with a 10-fold lower titre of Ad-Cre or Ad-Ctrl, with or without a single dose of TC. The combination of TC with low-titer Ad-Cre did not induce prolonged liver growth, as expected, but induced nodules at 4 months and advanced tumours at 8 months. In contrast, Ad-Cre activation of β-catenin induced only small nodules at 8 months ( Supplementary Fig. 6a ). Liver appearance and haematoxylin and eosin staining showed typical HCC structure in the 8-month TC plus Ad-Cre tumours ( Supplementary Fig. 6b,d ). Liver weight is increased at 4 months in both TC and TC plus Ad-Cre groups. At 8 months, large tumours in the TC plus Ad-Cre group greatly increased the liver weight. As in the heterozygous ctnnb1 wt/loxP(ex3) tumours, gene expression studies confirmed the induction of β-catenin target genes GS and Axin2 in both normal tissue and the tumours in the doubly activated livers, and the tumours also expressed known HCC markers. Gene expression in these tumours recapitulates that observed in the tumours induced in ctnnb1 wt/loxP(ex3) mice. CAR expression is reduced in liver tumours compared with non-tumour tissue and other groups ( Supplementary Fig. 7 ). CAR/β-catenin tumours model human HCC Database searches indicate that CAR is broadly expressed in human HCC, and global gene expression data in n =104 HCCs versus n =10 metastases to liver confirms that CAR mRNA is present in the vast majority of the HCC samples, but not in the metastatic tumours [42] . At the protein level, we observed human CAR expression in at least a subset of HCC ( Supplementary Fig. 8 ). Expression of CAR, like other liver markers, may decline as tumour stage advances. We used gene expression profiling to explore the potential human relevance of the CAR plus β-catenin tumorigenic pathway to the human disease. Cross-species comparison of the mouse tumour expression profiles with those from genotyped human HCC patients with or without alterations in β-catenin ( CTNNB1 ) revealed a unique gene expression signature present in both the mouse tumours and a subset of the human tumours. Strikingly, unsupervised clustering showed that this signature is found in the subset of human HCC with activating CTNNB1 mutations ( Fig. 7 ). The 82-gene signature includes 22 genes that have nearby CAR-binding sites identified by genome-wide binding studies that will be detailed elsewhere. The upregulated genes also include at least 10 known or candidate β-catenin targets, such as the ephrin receptor EFB2 (ref. 43 ) and the T-Box transcriptional repressor TBX3 (ref. 44 ), and also the Wnt pathway components LEF1 and TCF7. This conserved gene expression signature demonstrates that mouse tumours generated by the combined activation of CAR plus β-catenin model a unique subset of human HCC. 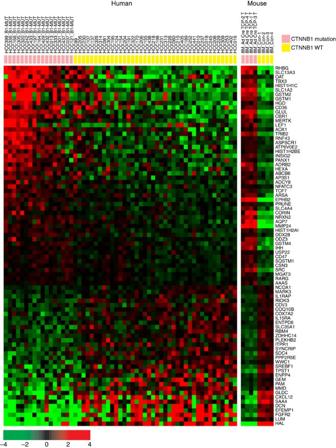Figure 7: Conserved gene signature between human HCC with CTNNB1 mutation and mouse HCC induced by TC (TCP) and β-catenin (Ad-Cre). Heat map of signature gene expression in human and mouse liver tumours. Eighty-two genes were significantly (P<0.001) associated in both data sets. Coloured bars at the top of the heat map represent CTNNB1 genotype and species as indicated (mouse wild-type CTNNB1 is normal liver). Figure 7: Conserved gene signature between human HCC with CTNNB1 mutation and mouse HCC induced by TC (TCP) and β-catenin (Ad-Cre). Heat map of signature gene expression in human and mouse liver tumours. Eighty-two genes were significantly ( P <0.001) associated in both data sets. Coloured bars at the top of the heat map represent CTNNB1 genotype and species as indicated (mouse wild-type CTNNB1 is normal liver). Full size image Dysregulated Wnt/β-catenin signalling is closely associated with human HCC [3] , [4] . However, activation of Wnt/β-catenin signalling alone does not induce spontaneous HCC in mouse models [5] , [6] , [7] , [8] , indicating that additional ‘hits’ are needed for tumorigenesis. In accord with this, liver tumours can be induced by the combination of β-catenin activation with other oncogenic inputs, including mutant H-ras [24] or heterozygous LKB1 (ref. 45 ) in mice, or carcinogen treatment of macaques [46] . β-catenin activation is also tightly associated with tumour promotion by PB, one of the best studied rodent models of hepatocarcinogenesis, since nearly all of the tumours induced by PB or other CAR activators carry activating mutations in β-catenin [17] , and the promotion effect of PB is lost in liver-specific β-catenin knockouts [22] . This strongly suggests a functional interaction between the oncogenic transcriptional coregulator and the nuclear xenobiotic receptor. Analysis of the β-catenin cistrome suggests that CAR may be a direct target [47] , which would be consistent with decreased CAR expression in the absence of hepatic β-catenin, and the modest increase we observed in response to β-catenin activation ( Supplementary Fig. 9 ). β-Catenin has also been reported to be a coactivator for other nuclear receptors [25] , [26] , suggesting another direct mechanism for functional synergy. However, several direct tests of effects of β-catenin on CAR, or vice versa, did not provide clear evidence for alterations in transactivation or expression levels ( Fig. 2 , Supplementary Fig. 1 ). More importantly, we did not observe significant effects of activation of either of the transcription factors on the other at the most basic level of direct target gene expression in vivo . Thus, their potent functional synergy cannot be attributed to simple, direct interactions or modulation of transcriptional output. Instead, our studies revealed a less direct, but more fundamental synergy in growth control. We found that chronic activation of Wnt/β-catenin alone induces senescence in the liver, as previously observed in the gut [10] and skin [12] , and demonstrated that CAR activation overcomes this block to β-catenin-induced growth. We showed previously that the CAR-dependent induction of Mdm2 is sufficient to block p53-dependent apoptosis in response to DNA damage [14] . Consistent with this, we found that CAR activation induces Mdm2 and FoxM1 to suppress β-catenin-induced growth inhibition. When combined with β-catenin activation, CAR activation reverses the induction of inflammatory markers, SA-β-galactosidase and expression of p53 and its downstream targets p21 and p27. We suggest that the rapid induction of Mdm2 in response to CAR activation prevents the ability of p53 to drive the later senescent response to β-catenin activation. The induction of FoxM1 and its downstream target Skp2 may also contribute to both this anti-senescent effect and CAR-induced growth. Thus, we and others have found that FoxM1 is an important mediator of CAR-induced liver cell proliferation [32] . FoxM1 is essential for the initiation of carcinogen-induced liver tumours, and its overexpression leads to the direct upregulation of proliferative genes such as Cdc25b, Cyclin D1, Cyclin B1, Polo-like kinase 1 and c-Myc [35] . Treatment with a FoxM1 inhibitor efficiently reduced proliferation and angiogenesis in a mouse model of HCC [48] . FoxM1 also induces expression of Skp2, a component of the ubiquitin ligase involved in proteasome-mediated degradation of cell cycle inhibitors, including p21 and p27. Consistent with this, p27 expression was increased when FoxM1 expression was decreased in the invasive HCC cell line MHCC-97H [49] . Although Cyp2b10 expression is lost, FoxM1 and Skp2 are also overexpressed in the tumours that result from long-term activation of CAR and β-catenin. A recent study indicated that Wnt signalling activates FoxM1, and that FoxM1 promotes β-catenin nuclear localization and modulates Wnt target gene expression in glioma [11] . Thus, FoxM1 could also contribute to β-catenin-positive HCC. In accord with the previous results, hepatic β-catenin activation also increased FoxM1 expression in the short term ( Fig. 3d ). However, the acute induction of FoxM1 in response to CAR activation was not sufficient to induce β-catenin nuclear localization. Our demonstration that the tumours induced by the combined activation of CAR and β-catenin in mice share an extensive gene expression signature with the β-catenin-activated subset of human HCC strongly supports the relevance of this model to the human disease. This is in direct contrast to suggestions that the rodent PB model is not relevant to human HCC, because epidemiologic studies generally do not show increased HCC incidence in human patients treated with PB or other anti-epileptic agents [50] although there is a potential outlier [51] . However, since PB by itself is a very poor carcinogen in rodents, its impact on hepatocarcinogenesis is dominated by the initiation-promotion model. Since this model is strictly dependent on the order of treatment, tumours should be increased only in the presumably quite small subset of patients exposed to carcinogens or mutagens shortly before PB treatment. Particularly, since the induction of hepatic drug metabolism could be expected to inactivate mutagens, the lack of a clear epidemiologic effect is not surprising, and does not preclude PB tumour promotion in humans. Overall, our results identify a quite unexpected route to hepatocyte expansion. The possibility of transient pharmacologic activation of both pathways, for example, via a specific human CAR agonist and either a Wnt ligand [52] or a synthetic β-catenin activator [53] , [54] , raises the prospect of therapeutic uses of this mechanism in the context of compromised liver function. Although we have observed appropriate responses of CAR and β-catenin target genes in preliminary studies, we have not observed either an initial senescent response to β-catenin activation or increased proliferative responses to double activation in primary hepatocytes ( Supplementary Fig. 10 ) or liver-derived cell lines. Our results also identify a novel, mutagen-independent liver tumour model that combines pharmacologic and genetic activation of two quite different transcriptional pathways. The clear association of these mouse tumours with β-catenin-activated HCC, which accounts for a significant fraction of human HCC [55] , [56] , makes this new model a powerful tool for tumour prevention and treatment studies with direct relevance to human HCC. Main reagents Ad5-CMV–GFP (cytomegalovirus–green fluorescent protein) or Cre virus was prepared by the Vector Development Laboratory at Baylor College of Medicine. The virus was diluted in Dulbecco’s phosphate-buffered saline (DPBS, Invitrogen) before tail vein injection. TC was purchased from Sigma-Aldrich and dissolved in corn oil. Animal maintenance and treatments Male mice starting at 10 weeks of age were used for all the experiments. Ctnnb1 loxP(ex3)/loxP(ex3) mice were kindly provided by Dr. Jeffery Rosen. To generate a mouse model, which has both activation of β-catenin and CAR, Ctnnb1 loxP(ex3)/loxP(ex3) mice were injected with high dose (10 9 p.f.u.) or low dose (10 8 p.f.u.) of Ad5-CMV-Cre virus via tail vein and intraperitoneally injected with TC (3 mg kg −1 body weight) at the same time. Mice were killed at different time points as indicated. Experiments involving mice were approved by the Institutional Animal Care and Use Committee of Baylor College of Medicine. Liver histology Livers were removed and pieces were fixed in 4% formaldehyde–PBS solution, embedded in paraffin, sectioned at 5 μm and stained with haematoxylin and eosin. For 2-bromodeoxy-uridine (BrdU)-staining, mice were injected intraperitoneally with the BrdU solution (10 mg kg −1 body weight) 2 h before being killed. Liver sections were prepared and stained using a BrdU labelling and detection kit (Roche). Immunohistochemistry was performed following the instruction of the procedure for each antibody. Sections prepared from the paraffin-embedded blocks were stained with β-catenin antibody (1:400), GS antibody (1:800) (BD transduction), Ki67 (1:500) (BD Pharmingen) and AFP (1:200) (kindly provided by Dr Milton Finegold). Detection of SA-β-gal activity was performed using the SA-β-gal staining kit (cell signalling). Ki67 and SA-β-gal positive cells were counted in three randomly selected fields for each sample, and each time point included sections from at least three mice. Serum parameters Before sacrifice, blood was collected from the orbital plexus and transferred into the Capiject Micro Collection Tubes (Terumo). Samples were centrifuged at 6,000 g for 10 min to separate serum. ALT levels were measured using the ALT reagent set (Teco Diagnostics). Bile acids levels were measured using the bile acid-L3 K assay kit (Diagnostic Chemicals). Cholesterol and triglyceride levels were determined by assay kits from Thermo DMA. Glucose was measured by Infinity glucose kit (Thermo Scientific). Quantitative real-time PCR Total RNA was isolated from livers using TRIZOL reagent. cDNA was prepared using superscript reverse transcriptase (Invitrogen). Gene expression was quantified by SYBR Green quantitative PCR using the ABI Prism 7500 sequence detection system (Applied Biosystems). The relative quantification analysis was performed by calculating the ratio of the mRNA amount of the gene of interest over the amount of internal control cyclophilin gene. Primer information can be provided upon request. Western blot Mice were killed at different time points as described. Liver tissues were removed, snap-frozen in liquid nitrogen and stored at −80 °C until use. For protein extraction, tissues were homogenized in a cold lysis buffer (50 mM Tris-HCl, pH 7.4; 1% NP-40; 0.5% sodium deoxycholate; 150 mM NaCl; 1 mM EDTA) containing protease and phosphatase inhibitor cocktails (Roche). After homogenization, the tissue lysates were allowed to solubilize for 1 h at 4 °C with rotation, and then were centrifuged at 19,700 g for 30 min at 4 °C. The supernatants were used for immunoblot analyses. Nuclear extract was performed by using nuclear and cytoplasmic extraction kit (Pierce). Western blots were performed following the procedure according to different antibodies. A total of 25 to 50 μg of protein was loaded for each lane and transferred to PVDF membrane. Protein expression was analysed by immunoblotting with β-catenin (Cell Signaling), phospho-β-catenin (Cell Signaling), β-actin (Cell Signaling), H3 (Cell Signaling), p21 (BD pharmingen), p53 (kindly provided by Dr Loning Fu), phospho-Yap (Cell Signaling), Yap (Cell Signaling), GS (BD Pharmingen). All dilutions are 1:1,000, except that H3 antibody dilution is 1:5,000 and GS antibody dilution is 1:3,000. Full gel scans are shown in Supplementary Fig. 11 . Microarray analysis Mouse liver samples (non-tumour and tumour) were collected and snap-frozen. Total RNA was extracted by using a mirVana RNA Isolation labelling kit (Ambion, Inc.). Five-hundred nanograms of total RNA were used for labelling and hybridization (mouse-6 BeadChip v.2 microarray, Illumina), according to the manufacturer’s protocols. After the bead chips were scanned with an Illumina BeadArray Reader (Illumina), the microarray data were normalized using the quantile normalization method in the Linear Models for Microarray Data package in the R language environment. The expression level of each gene was transformed into a log 2 base before further analysis. Using Illumina microarray platform (mouse-6, version 2), we collected gene expression data from eight livers of Ctnnb1 wt/loxP(ex3) and wild-type mice. We next identified genes whose expression is significantly associated with active mutation of Ctnnb1 and development of HCC in mouse by comparing gene expression data from HCC tissues from Ctnnb1 wt/loxP(ex3) mice with those from wild-type liver ( P <0.001 by two-sample t -test). Expression of 3,578 genes was significantly different when compared with normal mouse liver. Of note, since mouse HCC tissues with active Ctnnb1 mutation were compared with normal liver with wild-type Ctnnb1 , this large number of genes reflects the difference between HCC and normal liver in addition to the difference between active mutation of Ctnnb1 and wild type. Genes whose expression is significantly associated with active mutation of CTNNB1 in human HCC were also identified with the use of gene expression data from 57 HCC patients from INSERM cohort [57] . Expression of 1,313 genes was significantly ( P <0.001) associated with CTNNB1 mutations. Overlapped genes (82 genes) in two gene lists from human and mouse were further selected as evolutionarily conserved genes whose expression is significantly associated with active mutation of CTNNB1 and development of HCC in both human and mouse. Human HCC specimen analyses The frozen samples of human HCC were provided by the City of Hope National Medical Center, and the pathological description and analyses were performed by the pathologists in the Department of Pathology. All the tissues were accessed under a City of Hope National Medical Center Institutional Review Board protocol (IRB 06026) and informed written consent was obtained from all the subjects. The lysates of tumour and non-tumour adjacent tissues were prepared with the T-PER tissue Protein Extraction Reagent (Pierce). The CAR antibody was purchased from R&D and used as 1:1,000 dilution for the western blotting. Statistics Data presented in all the figures are mean±s.e. The number of subjects is indicated by n . Sample size was determined empirically on the basis of preliminary experiments to ensure appropriate statistical power. No samples were excluded and mice were randomly allocated to experimental groups before the start of treatments. Figures shown are representative of consistent results; differences between different genotypes were calculated by the two-tailed Student’s t -test. All statistical tests with P <0.05 were considered significant. One-way ANOVA analysis was used to determine the initial phenotype of liver weight/body weight ratio and proliferation. Two-way ANOVA analysis was used to determine the specific effect of two different stimuli (CAR activation versus β-catenin activation) on liver proliferation and senescence. In the attached tables, column factor is Ad-Co/Ad-Cre treatment, while row factor is Veh/TC treatment. Accession codes: Gene expression data have been deposited in the Gene expression Omnibus database with the accession code GSE43628 . How to cite this article: Dong, B. et al. Activating CAR and β-catenin induces uncontrolled liver growth and tumorigenesis. Nat. Commun. 6:5944 doi: 10.1038/ncomms6944 (2015).